The structure of superantigen complexed with TCR and MHC reveals novel insights into superantigenic T cell activation Superantigens (SAgs) are bacterial toxins that interact with immunoreceptors, T cell receptor (TCR) and major histocompatibility complex (MHC) class II, conventionally through the variable β-domain of TCR (TCRVβ). They induce a massive release of cytokines, which can lead to diseases such as food poisoning and toxic shock syndrome. In this study, we report the X-ray structure of the ternary complex between staphylococcal enterotoxin H (SEH) and its human receptors, MHC class II and TCR. The structure demonstrates that SEH predominantly interacts with the variable α-domain of TCR (TCRVα), which is supported by nuclear magnetic resonance (NMR) analyses. Furthermore, there is no contact between MHC and TCR upon complex formation. Structural analyses suggest that the major contact points to TCRVα are conserved among other bacterial SAgs. Consequently, a new dimension of SAg biology emerges, suggesting that in addition to the conventional interactions with the TCRVβ domain, SAgs can also activate T cells through the TCRVα domain. Staphylococcus aureus is one of the most formidable, disease-causing bacteria affecting humans. This bacterium causes numerous illnesses in humans, such as food poisoning, skin infections, toxic shock syndrome and autoimmune disorders. In particular, methicillin- and vancomycin-resistant strains of S. aureus are a medical challenge. S. aureus produces multiple toxins (SEA-U) at high nanogram to low microgram quantities, which has a major role in diseases caused by the bacteria [1] . The toxins produced are called superantigens (SAgs) because of their ability to activate large populations of human T cells, in contrast to conventional antigens [2] . SAgs simultaneously bind major histocompatibility complex (MHC) class II molecules on antigen-presenting cells and the T cell receptor (TCR) on T cells [3] . This crosslinking ultimately induces an overactive immune response and leads to the production of cytokines, such as tumour-necrosis factor-α, interleukin-2 and interferon-γ, which may result in toxic shock syndrome and other immune-mediated diseases [2] . The best-characterized bacterial SAgs are produced by S. aureus and by a related disease-causing bacteria, Streptococcus pyogenes . Bacterial genome sequencing has revealed that there is a large number of genetically distinct SAgs produced by these organisms, with more than 30 different serotypes [4] . S. aureus secretes the staphylococcal enterotoxins (SEs) and the toxic shock syndrome toxin-1 (TSST-1), whereas S. pyogenes secretes the streptococcal pyrogenic exotoxins (SPEs). The different SAgs can be classified into five distinct evolutionary groups (I–V). Although these toxins are believed to have a conserved tertiary structure, each group engages its immunoreceptors in structurally and functionally diverse ways. Staphylococcal enterotoxin H (SEH) is classified to evolutionary group III, yet SEH is the most deviating SE in this group [5] . The class III SAgs are suggested to crosslink MHC class II molecules through a low-affinity site, as well as a high-affinity zinc-dependent site. However, the crystal structure of SEH in complex with MHC class II demonstrate that SEH interacts with MHC class II, exclusively by the high-affinity site [6] . Nevertheless, low-affinity sites for MHC may be present in SEH, but not captured in the crystal structure. There is currently no available structural information regarding how group III SAgs engage TCRs, which may be a consequence of the expected low affinity between the class III SAgs and the TCRs. Previous structural studies of SAgs from other classes engaging the variable β-domain of TCR (SEB, SEC 2−3 , SEK, TSST-1, SPE-A and SPE-C) use only the single β-chain of TCR [7] , [8] , [9] , [10] , [11] , and often, there are mutations in the TCR or SAg. To date, there is one report on structural studies of an SAg from mycoplasma ( Mycoplasma arthritidis mitogen, MAM) in complex with TCR and MHC, showing specific contacts between the SAg and both variable α-domain of TCR (TCRVα) and variable β-domain of TCR (TCRVβ). However, no previous study has yet described the ternary complex between a bacterial SAg secreted from S. aureus or S. pyogenes and both its receptors MHC class II and TCR. In this study, we have crystallized the ternary complex between the class III SAg, SEH and its human receptors MHC class II and TCR and elucidated the structure. The ternary complex structure is determined at 2.3 Å resolution. In addition, we have crystallized and determined a structure of the SEH–TCR complex at 2.1 Å resolution. Furthermore, a novel approach to study the interface interactions between SAgs and its immunoreceptors is by using nuclear magnetic resonance spectroscopy (NMR), as the affinities between the putative complexes are in many cases optimal for NMR analyses. In this study we have, in addition to the crystal structure, characterized the binding interfaces between SEH and TCR in solution using NMR. The combined data from NMR and X-ray crystallography clearly demonstrate that SEH predominantly binds to the TCRVα. Moreover, important residues in the interface between SEH and TCRVα were identified as conserved amino acids among many other structurally related SAgs. The overall structure of the TCR–SEH–MHC complex We determined the crystal structure of the ternary complex, including human MHC class II, human leukocyte antigen (HLA-DR1), binding the Influenza hemagglutinin (HA) (306–318) peptide (PKYVKQNTLKLAT), the human TCR (JM22:TRAV27/TRBV19) specific to the Influenza matrix protein (MP) (58–66) peptide (GILGFVFTL) and the bacterial SAg, SEH at 2.3 Å resolution. 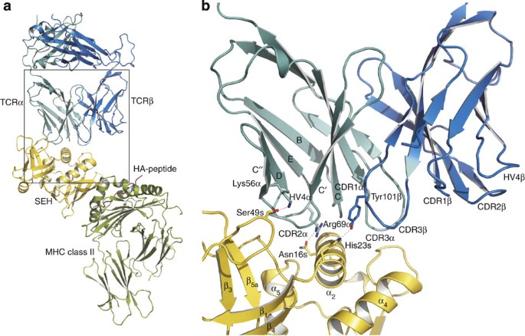Figure 1: The ternary X-ray structure of the TCR–SEH–MHC complex. (a) Ribbon representation of the overall structure, with the TCRα and β-chains coloured in cyan and blue, respectively, SEH coloured yellow, MHC class II coloured green and the HA-peptide in red. TCR binds mainly with its Vα domain to the so-called 'TCR binding cleft' of SEH. (b) Close-up view of the interaction interface between TCR and SEH with hydrogen bonds shown as dotted lines. Secondary structure elements of SEH and TCR are labelled according to standard. In the asymmetric unit, there is one copy of each protein, and the complex packs in the space group C2 ( Table 1 ). In addition, we solved a high-resolution structure including only the TCR and SEH at 2.1 Å resolution ( Table 1 ). TCR and MHC were both expressed in E. coli as inclusion bodies and refolded, according to earlier published protocols [12] , [13] , [14] . SEH was expressed in the periplasm of E. coli as earlier described by Nilsson et al . [15] The proteins were mixed in an equimolar ratio and the crystals were formed in a few weeks. The ternary complex has an extended overall structure, with the SEH binding mainly to the TCRVα part of the TCR and on top of the MHC class II through the β-chain ( Fig. 1a ). The contact area between SEH and MHC is 1465 Å 2 , which correlates well with the previously published SEH–MHC structure [6] . The buried surface area between SEH and TCR is 1369 Å 2 , where TCRα contributes to 94% and TCRβ to 6%. Upon ternary complex formation, contacts between MHC class II and TCR are completely prevented ( Fig. 1a ). In the ternary structure, we have modelled residues 2–200 in TCRα, 3–244 in TCRβ, 4–181 in MHCα, 2–189 in MHCβ, 1–13 in the Influenza HA peptide and 1–215 in SEH. Moreover, there are 280 water molecules and 4 glycerol molecules in the structure. In the high-resolution structure, including only TCR and SEH, we could model residues 2–200 in TCRα, 3–243 in TCRβ and 1–215 in SEH, along with 249 waters and 3 glycerol molecules. The SEH–TCR structure also crystallized in the space group C2 and each asymmetric unit contains one copy of the SEH–TCR complex. The buried surface area between SEH and TCR is 1487 Å 2 , where TCRα contributes to 83% and TCRβ to 17%. Furthermore, the two structures (ternary complex and SEH–TCR structure) are highly similar ( Fig. 2a ), with a total root mean square deviation (RMSD) of 1.2 Å calculated using secondary structure matching (SSM), where differences in the TCRβ chain contribute the most. Table 1 Data collection and refinement statistics. Full size table Figure 1: The ternary X-ray structure of the TCR–SEH–MHC complex. ( a ) Ribbon representation of the overall structure, with the TCRα and β-chains coloured in cyan and blue, respectively, SEH coloured yellow, MHC class II coloured green and the HA-peptide in red. TCR binds mainly with its Vα domain to the so-called 'TCR binding cleft' of SEH. ( b ) Close-up view of the interaction interface between TCR and SEH with hydrogen bonds shown as dotted lines. Secondary structure elements of SEH and TCR are labelled according to standard. 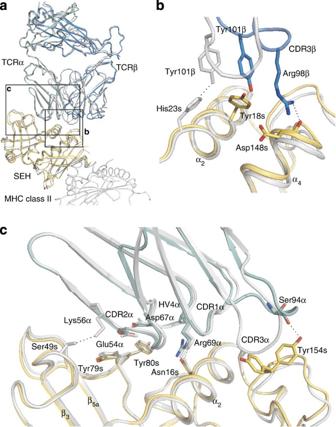Figure 2: Superposition of the SEH–TCR structure on the ternary TCR–SEH–MHC structure. (a) Ribbon representation of the overlay between the two structures (the binary structure is coloured cyan, blue and yellow, and the ternary structure grey). (b) Close-up view of the interaction between TCRVβ and SEH in the two complexes. Hydrogen bonds are marked with dotted lines. (c) Close-up view of the interface between TCRVα and SEH. Important residues are shown as sticks and hydrogen bonds marked as dotted lines. Tyr154s is refined with a dual conformation, where the one engaged in hydrogen bonding has occupancy 0.4. Full size image Figure 2: Superposition of the SEH–TCR structure on the ternary TCR–SEH–MHC structure. ( a ) Ribbon representation of the overlay between the two structures (the binary structure is coloured cyan, blue and yellow, and the ternary structure grey). ( b ) Close-up view of the interaction between TCRVβ and SEH in the two complexes. Hydrogen bonds are marked with dotted lines. ( c ) Close-up view of the interface between TCRVα and SEH. Important residues are shown as sticks and hydrogen bonds marked as dotted lines. Tyr154s is refined with a dual conformation, where the one engaged in hydrogen bonding has occupancy 0.4. Full size image Overall, the structural rearrangements upon complex formation are rather small; hence, the different proteins included in the complex are analogous with the uncomplexed structures [16] , [17] , [18] . SEH has an N-terminal OB-fold comprising of the β-strands β 1 –β 5 and one α-helix (α 3 ). The C-terminal domain, consisting of a large β-sheet (β 6 , β 7 , β 9 , β 10 and β 12 ) and three α-helices (α 2 , α 4 and α 5 ), forms a β-grasp motif. The HLA-DR1 class II MHC is made up of two parts (MHCα and MHCβ), each including an immunoglobulin domain and an α-helix packed against a large β-sheet, with the HA-peptide bound between the two helices. The TCR consists of two chains (an α- and a β-chain) each including two immunoglobulin domains. The chains have one constant and one variable domain, with the constant domains kept together by an introduced disulphide bridge between Cys158α and Cys171β [12] (residues belonging to TCRα, TCRβ, and SEH will be designated with α, β or s). The loops in the two variable domains contact the antigen in a conventional immune response, but are known to contact the SAg as well. There are four of these loops in each domain, which are abbreviated as CDR1–3 and HV4. In line with the earlier published SEH–MHC structure (1HXY), SEH binds to MHC with its large, C-terminal β-sheet in a very similar manner as was described by Petersson et al . [6] However, there is no Zn 2+ ion present in the structure described here, in contrast to the structure reported by Petersson et al . [6] This is likely due to difficulties in crystallization in the presence of zinc. However, all contacts between SEH and peptide-MHC are conserved in the interface and hence are enough to create a stable complex formation in the crystal. In addition, Fernandez et al . [19] have earlier reported on low occupancy for zinc in the SEI–MHC class II complex. Thus, in both these cases, zinc is most likely important for complex formation in solution, but not essential in the crystalline form, as the conserved hydrogen bonds between SAg and peptide-MHC are enough to promote crystal packing. SEH binds mainly to TCRVα The TCR binds to SEH mainly through its TCRVα domain ( Fig. 1b ) using the same cleft in SEH, the so-called 'TCR binding cleft', as the TCRVβ uses when binding other SAgs, for example, SEB (Fig. 6b) [9] . The contact points from TCR are predominantly the CDR2α loop and the HV4α loop. In addition, there are minor contributions from the CDR1α and CDR3α loops. There are only two hydrogen bonds between SEH and TRAV27, Arg69α in the HV4 loop to Asn16 s and from Lys56α in the C″ strand to Ser49 s ( Fig. 1b , Supplementary Table S1 ). However, a third hydrogen bond is seen only in the SEH–TCR structure between Ser94α and Tyr154 s ( Fig. 2c , Supplementary Table S1 ), but Tyr154 s was refined with two alternative conformations and only the second conformation, with occupancy of 0.4, is hydrogen bonding to Ser94α. Hence, the contact is not essential for complex formation. In the SEH–TCR structure, the hydrogen bond between Ser49 s and Lys56α is not seen, likely due to the flexibility of lysine residues. Moreover, a number of residues make van der Waals (vdW) contacts between SEH and TCR to contribute to the binding ( Supplementary Table S1 ). The main contacts are with residues from the TCRVα CDR2 loop (seven vdW contacts) and the HV4α loop (four vdW contacts), with the exceptions of Val28α in the CDR1α loop, Ser94α in the CDR3α loop and Val55α in the C′ strand ( Fig. 3a , Supplementary Table S1 ). There is a hydrophobic patch in SEH consisting of Tyr79 s and Tyr80 s, with their side chains pointing in opposite directions ( Fig. 3a and b ). Tyr79 s is making extensive vdW contacts to Gly52α, Gly53α and Glu54α in the CDR2α loop region, whereas Tyr80 s contacts the backbone oxygen of Gly52α in CDR2α as well as the side chain of Asp67α in HV4 ( Supplementary Table S1 ). Furthermore, a putative ion is bound to the main chain oxygens of His23 s and Ser77 s, as well as the side chain oxygen of the serine ( Fig. 4 , Supplementary Table S1 ). There are three water molecules contributing to the sixfold coordination of the ion that is positioned in the interface between SEH and the TCRVα. Its biological relevance remains unclear, but one of the water molecules makes a hydrogen bond to the side chain oxygen of Thr51α, likely contributing to the affinity of the complexes. In addition, the putative ion is present in both the ternary complex structure and the SEH–TCR structure, despite differing crystallization conditions; hence, it seems important for stable complex formation. Although SEH makes extensive contacts to TCRVα, there are also contacts to the TCRVβ chain, through the side chain of His23 s that is packed against the side chain of Tyr101β, and forming a hydrogen bond ( Figs 1b and 3c ). However, the hydrogen bond can only be seen in the ternary structure, and not in the SEH–TCR structure, suggesting flexibility in this region ( Fig. 2b ). In the binary structure, Tyr101β forms vdW contacts with Tyr18 s instead ( Fig. 2b , Supplementary Table S1 ). Furthermore, in the SEH–TCR structure, there is a hydrogen bond between Arg98β and Asp148 s ( Fig. 2b , Supplementary Table S1 ). 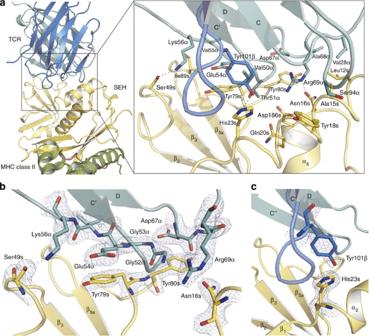Figure 3: The interface between SEH and TCR showing van der Waals contacts and hydrogen bonding. (a) TCRVα is shown in cyan, TCRVβ in blue and SEH in yellow. Amino acids involved in the contact are shown as sticks. The three hydrogen bonds are marked with dotted lines. (b) A 2Fo-Fcelectron density map (cutoff at 1.6σ) shown around residues in TCRVα and SEH that is most important for the interaction. (c) Electron density map (2Fo-Fc, cutoff at 1.6σ) shown around residues in TCRVβ and SEH involved in the binding. Figure 3: The interface between SEH and TCR showing van der Waals contacts and hydrogen bonding. ( a ) TCRVα is shown in cyan, TCRVβ in blue and SEH in yellow. Amino acids involved in the contact are shown as sticks. The three hydrogen bonds are marked with dotted lines. ( b ) A 2F o -F c electron density map (cutoff at 1.6σ) shown around residues in TCRVα and SEH that is most important for the interaction. ( c ) Electron density map (2F o -F c , cutoff at 1.6σ) shown around residues in TCRVβ and SEH involved in the binding. 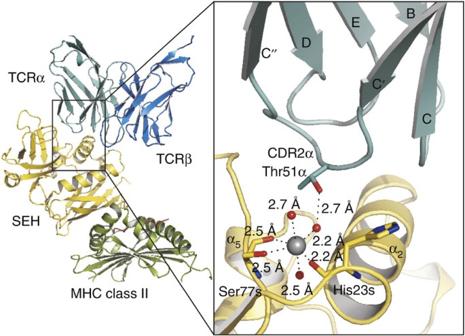Figure 4: The putative metal ion site in the SEH–TCR interface. A putative metal ion, modelled as Na+in the crystal structures, is found in the interface between SEH and TCRVα. Two residues from SEH (Ser77s and His23s) and three water molecules are coordinating the metal ion. Furthermore, one of the coordinating water molecules forms an additional hydrogen bond to Thr51α in TCRVα. Full size image Figure 4: The putative metal ion site in the SEH–TCR interface. A putative metal ion, modelled as Na + in the crystal structures, is found in the interface between SEH and TCRVα. Two residues from SEH (Ser77s and His23s) and three water molecules are coordinating the metal ion. Furthermore, one of the coordinating water molecules forms an additional hydrogen bond to Thr51α in TCRVα. 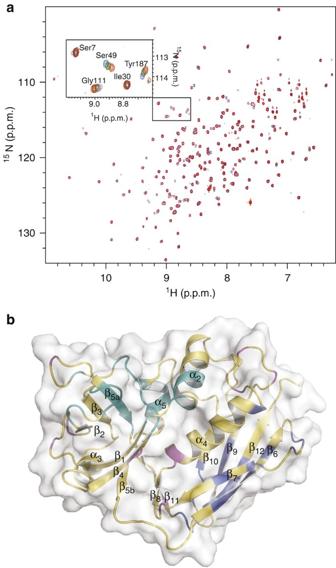Figure 5: Chemical shift perturbations detected by NMR after addition of TCR to SEH. (a) The 2D (1H,15N) HSQC spectrum of 120 μM SEH (red) and in the presence of 21 μM TCR (blue). Inset: The SEH protein is titrated with TCR at increasing TCR:SEH stoichiometry. Red: 0, orange 1:20, green: 1:10, blue: 1:6. The superimposed inset shows that the signals from Ser7s and Ile30s do not change during the titration, whereas the signals from Ser49s, Tyr187s and Gly111s are markedly affected. (b) Chemical shift perturbations mapped on the crystal structure of SEH. The primary TCR binding site is coloured in cyan, the secondary putative site is shown in blue, and residues not clearly belonging to any site are coloured pink. Full size image Complex formation in solution In Figure 5 , the 2D ( 1 H, 15 N) HSQC spectrum of the SEH protein at 900 MHz is shown ( Fig. 5a ). The spectrum is well dispersed and most peaks are resolved. The sequential assignment of the SEH protein was reported elsewhere [20] . According to the chemical shift index, the structural integrity of the SEH protein in solution shows no deviation from the reported crystal structures [16] , [20] . An NMR study of the transient interaction between SEH and the TCR was performed. Several 2D ( 15 N, 1 H) HSQC spectra were recorded in a titration series at increasing TCR:SEH ratios, to a final ratio of 1:6. During the titration, several peaks shifted or broadened in the NMR spectra ( Fig. 5a ). In Supplementary Table S2 , the 20% of the SEH peaks exhibiting the largest changes in chemical shifts and/or intensities are shown ( Supplementary Table S2 ). The changes are essentially localized to surface-exposed amino acids in two separate well-defined regions (coloured cyan and blue, Fig. 5b ) and not distributed over the entire protein. Hence, the NMR titration demonstrates the overall structural integrity of SEH on binding to the TCR. The first region of SEH (cyan in Fig. 5b ), exhibiting changes in peak positions or intensities, corresponds to the binding site of the TCR captured in the crystal structure. This region includes residues 17–25 in the α 2 -helix of SEH, residues 44–50 in a loop region between β 2 and β 3 strands, residues 75–81 and 84 in the loop region between β 4 and β 5a , residues 91–94 of the β 5a strand and residues 182 and 187–191 of the α 5 -helix ( Fig. 5b ). Figure 5: Chemical shift perturbations detected by NMR after addition of TCR to SEH. ( a ) The 2D ( 1 H, 15 N) HSQC spectrum of 120 μM SEH (red) and in the presence of 21 μM TCR (blue). Inset: The SEH protein is titrated with TCR at increasing TCR:SEH stoichiometry. Red: 0, orange 1:20, green: 1:10, blue: 1:6. The superimposed inset shows that the signals from Ser7s and Ile30s do not change during the titration, whereas the signals from Ser49s, Tyr187s and Gly111s are markedly affected. ( b ) Chemical shift perturbations mapped on the crystal structure of SEH. The primary TCR binding site is coloured in cyan, the secondary putative site is shown in blue, and residues not clearly belonging to any site are coloured pink. Full size image The second region that exhibits chemical shift changes is located in the C-terminal domain of SEH (coloured blue) ( Fig. 5b ). This region comprises residues that are more scattered in the sequence but structurally are located around His206 s, which is one of the zinc coordinates in the complex structure between SEH and MHC ( Fig. 5b ) [6] . Hence, it is likely that the MHC class II would block binding of TCR to this site in vivo . Both the chemical shift changes and the exchange broadening of NMR signals can be used to analyse the kinetic properties of the complex. Results presented in Supplementary Table S2 reflect three cases: (1) changes only in chemical shifts, (2) changes in both peak positions and intensities, (3) changes only in intensities. Numerical simulations using McConnell equations for the concentrations used, assuming a dissociation constant ( K d ) of 10 μM and subdiffusion limited on-rate, show that the observed results are consistent with the medium to slow exchange process in the NMR time scale. Cases 1–3 correspond to small to large difference between the signal positions in the free and complex form of SEH. The exchange data may reflect several molecular processes, from full complex formation to an allosteric effect of localized conformational transitions in a protein structure unleashed by the complex formation. For SEH in solution, we see a picture, which is consistent with the complex interface observed in the crystal structure. Additional effects at the distant site near His206 s may point to a secondary binding site, whose relevance for the SEH–TCR function is unclear. Conserved residues are important for the contact with TCRVα It was discovered over 20 years ago that SAgs activate T cells by specific interaction with the TCRVβ domain [21] . Since then, many studies have confirmed these findings and this was recently reviewed by Fraser and Proft [22] . However, SEH is different as it binds and activates T cells through the TCRVα [23] , [24] . When comparing the SEH–TCR complex with other SAg–TCR structures that are available in the RCSB Protein Data Bank (SEB, SEC 3 , SEK, SPE-C, SPE-A, TSST-1), it is clear that TRAV27 binds SEH in the opposite direction compared with how TCRVβs recognize SAgs ( Fig. 6a ). Despite the TCRVα being rotated 180 °C compared with TCRVβ, it still binds the homologous cleft of SEH that the TCRVβ contacts in the other SAgs ( Fig. 6b ). TSST-1, however, represents a third way of binding TCR by the S. aureus and S. pyogenes SAgs, using a unique TCR engagement were the TCR is tilted compared with the other SAg–TCRVβ complexes [10] . The three major contact areas between SEH and TRAV27 are the two hydrogen bonds (Asn16s-Arg69α and Ser49s-Lys56α), and the hydrophobic patch in the middle of the TCR binding cleft of SEH ( Fig. 3b ). Interestingly, the hydrogen bond from Asn16 s to the TCR is conserved in four other SAg–TCR structures (SEB, SEC 3 , SEK and SPE-A), irrespective of whether the binding is to TCRVα or TCRVβ ( Fig. 7a ). In addition, Asn16 s is very well conserved among the S. aureus and S. pyogenes SAgs ( Fig. 7c ). Furthermore, the hydrophobic patch on SEH (Tyr79s/Tyr80 s) is also rather well conserved among other SAgs and seems to be important for the general contact with TCR ( Fig. 7a ). Hence, the structure of SEH in complex with TCR first suggests that there are two important handles on the SAgs that the TCR recognizes, and second that TCRVα and TCRVβ utilize the same way of binding, but in the opposite direction. This opens up the possibility of that SAgs, other than SEH, may bind TCR through the TCRVα domain, in addition to contacts with the TCRVβ domain. 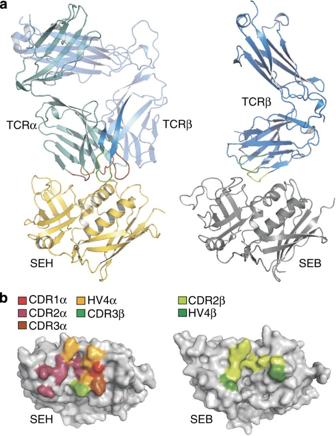Figure 6: Structural comparisons between SEH and SEB binding to TCRVα and TCRVβ, respectively. (a) SEH-TCRα (yellow and cyan) and SEB-TCRβ (grey and blue) shown as ribbon representation, illustrating the difference in binding orientation. (b) Surface representation of superimposed SEH and SEB, with the TCR binding areas marked in colours corresponding to the contacting CDR or HV loop, demonstrating that approximately the same surface of the SAg is used upon binding. Figure 6: Structural comparisons between SEH and SEB binding to TCRVα and TCRVβ, respectively. ( a ) SEH-TCRα (yellow and cyan) and SEB-TCRβ (grey and blue) shown as ribbon representation, illustrating the difference in binding orientation. ( b ) Surface representation of superimposed SEH and SEB, with the TCR binding areas marked in colours corresponding to the contacting CDR or HV loop, demonstrating that approximately the same surface of the SAg is used upon binding. 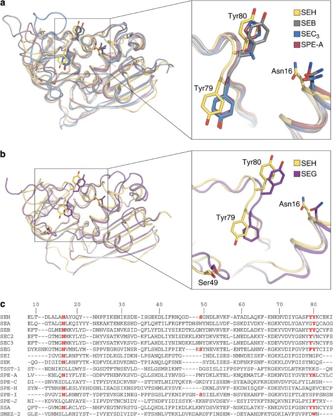Figure 7: Structural comparisons of SEH with other SAgs. (a) Structural alignment of SEB (grey), SEC3(blue) and SPE-A (red) with SEH (yellow), which have been cocrystallized and structurally determined with TCRβ. Asn16 of SEH is structurally conserved among all of these SAgs and is involved in TCR binding. Furthermore, the hydrophobic patch consisting of Tyr79 and Tyr80 in SEH is also preserved among most SAgs. (b) Structural alignment of SEH (yellow) and SEG (purple), showing the structural similarity. All of the crucial residues for TCR binding in SEH are conserved in SEG, apart from Tyr79, which corresponds to a phenylalanine instead. (c) Structural alignment of the crystal structures of several SAgs. Residues corresponding to Asn16, Ser49, Tyr79 and Tyr80 are marked in red. Full size image Figure 7: Structural comparisons of SEH with other SAgs. ( a ) Structural alignment of SEB (grey), SEC 3 (blue) and SPE-A (red) with SEH (yellow), which have been cocrystallized and structurally determined with TCRβ. Asn16 of SEH is structurally conserved among all of these SAgs and is involved in TCR binding. Furthermore, the hydrophobic patch consisting of Tyr79 and Tyr80 in SEH is also preserved among most SAgs. ( b ) Structural alignment of SEH (yellow) and SEG (purple), showing the structural similarity. All of the crucial residues for TCR binding in SEH are conserved in SEG, apart from Tyr79, which corresponds to a phenylalanine instead. ( c ) Structural alignment of the crystal structures of several SAgs. Residues corresponding to Asn16, Ser49, Tyr79 and Tyr80 are marked in red. Full size image SAgs are disease-causing bacterial toxins that are capable of interfering with the human immune system by crosslinking the TCR and MHC class II. In this way, they activate large numbers of T cells and hence elicit a very strong immune response. There are several structural reports on how SAgs from S. aureus or S. pyogenes engage the TCRVβ or the MHC class II, but there are no ternary complex structures available for SAgs from these disease-causing bacteria. We have for the first time crystallized and determined the structure at 2.3 Å of the complex between the full-length extracellular domains of TCR (TCRα and TCRβ), the SAg SEH and the extracellular part of the MHC class II molecule (including α- and β-chain and the bound HA-peptide). The complex structure clearly demonstrates that the main interaction between the TCR and the SAg is through the TCRVα (TRAV27). This is the first time that structural studies showing that a SAg from S. aureus predominantly binds to the TCRVα domain. In line with this structural result, the biological functions of SEH have earlier been studied in biochemical as well as cell-based assays, and both studies strongly suggest that SEH binds and activates T cells through the TCRVα domain [23] , [24] . The only available structural data of SAg in complex with both its immunoreceptors (full-length MHC and the variable chains of TCR) is a SAg from mycoplasma, MAM [25] . MAM has a completely different three-dimensional fold compared with the structurally studied SAgs from S. aureus and S. pyogenes [26] . MAM interacts with both the TCRVα and the TCRVβ, where TCRVβ accounts for roughly two-thirds of the buried surface area [25] . As the structure of MAM differs significantly from SEH, it is difficult to compare the two structures in a constructive manner. The variable domains of the TCRs in the TCR–MAM–MHC structure (2ICW) and the TCR–SEH–MHC (2XN9) were superimposed ( Supplementary Fig. S1 ) and interestingly, the two SAgs (MAM and SEH) bind in completely different orientations with almost no overlap. Furthermore, previous structural studies on the interactions between SAgs and their immunoreceptors have only been performed using the technique X-ray crystallography. Although X-ray crystallography is often the optimal method to use when studying specific interactions between proteins, the protein complexes are captured in a static position. Hence, to confirm that the complex formation occurs in solution, NMR is the more favourable technique to use. For the first time, NMR analyses have confirmed the specific binding between the TCR and a SAg. 15 N HSQC spectra of the free and the bound SEH molecule were compared, and residues showing chemical shift differences or extensive line broadening upon complex formation were denoted as significant in the interaction. The combined use of chemical shift changes and line broadening allows a better qualitative comparison of the solution and crystal complexes. The residues 13 and 17, adjacent to the hydrogen bonding Asn16 s, do not exhibit chemical shift changes upon complex formation, but for both residues, a significant line broadening occurs. The appearance of broadening without significant change in a signal position is an indication of an exchange process in the slow NMR time scale, which means largest difference in the peak position between the free and bound form of SEH. Although our NMR data are not amenable to a detailed quantitative analysis of the exchange process, the emerging picture is clear and gives a consistent view of the kinetics of the complex formation. It is consistent with the earlier reported K d in the micromolar range and the on-rate somewhat slower than the diffusion limited value of 10 8 M −1 s −1 . Hence, the solution NMR results strongly support the interactions that are seen in the crystal structure. The NMR analysis also suggests a second interaction site, distant from the SEH–TCR interface in the crystal complex. Despite localization close to the zinc-coordinating His206s, it is unlikely that the observed spectral changes are due to a concomitant titration of zinc or pH changes, as the pH was carefully monitored. Instead, it is more likely that the second site also takes part in an interaction with the TCR. SEH has evolved to expose two different interaction surfaces, and it cannot be ruled out that these surfaces enable a less specific, weaker interaction. However, it should be kept in mind that the second interaction surface overlaps with the high-affinity MHC class II binding site, so that it is possibly blocked from binding in an in vivo situation. In conclusion, this evidently shows the advantages of using NMR analyses to complement X-ray crystallography and also demonstrates a model system that can be utilized to study the activation mechanism by SAgs through the TCR. A characteristic hallmark for all SAgs has been TCRVβ-restricted activation of T cells [22] . Structural alignment among the SE and the SPE family suggest that amino acids in SEH, which are important for the contact to TRAV27 (Asn16s and the hydrophobic patch, Tyr79s and Tyr80s), are rather well conserved within the family ( Fig. 7c ). Explicitly, nearly all structurally determined bacterial SEs have a corresponding aspargine to Asn16s in the nearby region ( Fig. 7c ). Moreover, to date there are six unique publicly available X-ray structures of SAgs in complex with TCRVβ, and four of them use the correlating asparagines to contact the TCRVβ and three of them use the correlating hydrophobic patch to contact the TCRVβ. Thus, bacterial SAgs seem to be able to use the same contact mode when binding either TCRVα or TCRVβ, although the TCR domain has been rotated 180 °C ( Fig. 6a ). This raises a crucial biological question; can other bacterial SAgs also engage TCR through the TCRVα in this manner? The interaction between T cells and previously characterized SAgs is governed by the TCRVβ repertoire, but skewed TCRVα repertoires after stimulation with SEA, SEB, SEC or SEE have been detected [27] , [28] , [29] , [30] . This might be an indirect result, as variable α-domain specificity can be induced by the direct interaction between TCR and MHC class II [27] , [28] , [29] , [30] . However, recently it was reported that TRAV26 was significantly upregulated after SEB stimulation [31] . Likewise, all structural studies of TCR recognition by bacterial SAgs has only included the TCRVβ domain; hence, any putative contacts between the SAgs and the TCRVα would not be possible to detect. Taken together, this implies that this novel feature of SEH, T cell activation through the TCRVα domain, is not unlikely to be exhibited by other SAgs. Structural alignment among bacterial SAgs suggests that SEG in particular has amino acids strikingly similar to those in SEH responsible for the TCRVα contact ( Fig. 7b ). SEG and SEB belongs to group II SAgs, which has been classified to engage TCRVβ through mostly conformation-dependent mechanisms that are largely independent of specific TCRVβ amino-acid side chains [5] . Thus, SAgs in group II seem to have rather broad specificity for TCR, which may also include interactions with the TCRVα domain. This is in contrast to SAgs belonging to group IV, for example, SPE-C, where the crystal structure of SPE-C–TCRVβ shows multiple contacts with both side-chain and main-chain atoms of TCRVβ and that all three CDR loops were engaged, as well as the HV4 region [11] . Also, SPE-C does not have any correlating amino acids to those that are responsible for the contact between SEH and TCRVα. Hence, it is rather unlikely that SAgs such as SPE-C would bind TCRVα. In conclusion, here we have shown the manner in which SEH binds TCR and suggest that it is not unlikely that SAgs belonging to either group II or group III (for example, SEB or SEH) can also activate T cell in a TCRVα-restrictive manner, whereas SAgs belonging to group IV may not have a broader specificity for the TCR, than was earlier discovered. In addition to the important information regarding the nature of such a potent T cell stimulus as SAgs, the finding presented here have vital implications for future strategies in designing drugs aimed to prevent or interfere with the interactions between SAgs and the host receptors. One important consequence is that investigating whether a patient has a skewed variable β-domain repertoire, which is a common way to determine whether a disease is caused by SAg or not [32] , [33] , [34] , may be misleading, as our results show that Vβ interaction is not the exclusive means of T cell activation by SAgs. Thus, the results presented here, describing the previously unknown feature of SAgs, activation of T cells through the TCRVα, could have significance for the understanding of these diseases. Hence, the findings are the key to understanding the nature of SAg-mediated T cell activation, and also have central implications for future strategies aimed at preventing or modulating the often pathogenic response to SAgs. Protein expression and purification Unlabelled SEH was produced in E. coli K12 strain UL635 in line with methods published earlier [15] , and SEH labelled with NMR active isotopes were produced in line with methods described by Saline et al . [20] Briefly, the protein was overexpressed in E. coli . Following isolation of the periplasmic protein fraction, SEH was subjected to cationic exchange chromatography (Resource S 6-ml column, GE Healthcare) on an ÄKTA explorer (GE Healthcare). For crystallization purposes, SEH was further purified by size exclusion chromatography (Superdex 75 10/300 GL column, GE Healthcare). Back exchange of amide protons of the triple-labelled NMR sample was performed in a shaking incubator (600 r.p.m., 50 °C, 60 h). A total amount of 2 mg triple-labelled SEH was brought to a final concentration of 0.8 mM (in 300 mM NH 4 OAc pH 6.8, 150 mM NaCl, 90:10 H 2 O/D 2 O) in a 3-mm Shigemi tube (100 μl). Double-labelled sample was concentrated to 1.6 mM (in 10 mM TRIS, pH 7.0, 40 mM NaCl, 90:10 H 2 O/D 2 O) in a 5-mm Shigemi tube (300 μl) and single-labelled SEH was in 10 mM TRIS, pH 7.0, 40 mM NaCl, 90:10 H 2 O/D 2 O with varying concentrations. The soluble human TCR (JM22:TRAV27/TRBV19) specific to the Influenza matrix protein (MP) (58–66) peptide (GILGFVFTL) was produced as disulphide-linked αβ heterodimers, as previously published [12] , [14] . E. coli BL21(DE3) cells harbouring the α- and β-chain plasmids were grown separately. Inclusion bodies were collected and washed before refolding. The latter was carried out by dialysis, and purification of refolded protein was done by anion exchange chromatography (Resource Q 6-ml column, GE Healthcare), followed by size exclusion chromatography (Superdex 75 10/300 GL, GE Healthcare). The MHC class II HLA-DR1 (α-chain DR*0101 and β-chain DRB1*0101) was produced as described earlier [13] , apart from minor changes. Chains were grown separately in E. coli , and inclusion bodies were collected from the lysate. These were washed and purified by anion exchange chromatography (Resource Q 6-ml column, GE Healthcare). Refolding was carried out by dilution of the chains to a final concentration of 0.08 μM in the presence of HA(306–318) peptide (PKYVKQNTLKLAT) from Influenza HA, and further purification was carried out by anion exchange chromatography (Resource Q 6-ml column, GE Healthcare). Crystallization Proteins were mixed in an equimolar ratio to a final concentration of 7 and 11 mg ml −1 of SEH–TCR and TCR–SEH–MHC, respectively, and filtered in a Vivaclear clarifying filter 0.8 μm (Sartorius). Crystals of the SEH–TCR complex grew in 11.5% (w/v) PEG 5000 MME, 0.1 M MES, pH 6.5 and 0.1 M NaCl at 20 °C, while the ternary complex crystallized in 15% (w/v) PEG 5000MME, 0.1 M BIS-TRIS, pH 7.0 and 0.1 M NaCl at 4 °C. Before flash freezing in liquid nitrogen, crystals were soaked in 20% (v/v) glycerol for cryo protection. Data were collected at the ESRF beamlines ID 14–1 and 14–2 at 100 K and at a wavelength of 0.933 Å. Structure determination and refinement Initial processing of the ternary complex data was carried out with Mosflm [35] , and subsequent scaling and molecular replacement was performed with the CCP4 package [36] . Scaling and merging was carried out with Scala, where 5% of the data were chosen as a subset for calculation of free R-values. For molecular replacement using Phaser [37] , models of the MHC α- and β-chains, and SEH were generated from the structure 1HXY [6] , whereas TCR α- and β-chains were extracted from 1OGA [18] , and all protein chains were allowed to locate irrespectively to each other. Several rounds of manual model building in Coot [38] and restrained refinement in Refmac5 (ref. 39 ) were carried out. The HA-peptide was built manually into the density. For validation, a composite omit map, omitting 10% of the structure, was calculated with CNS [40] . For the SEH–TCR complex, data were processed using XDS [41] , whreas subsequent refinement was carried out in the same way as for the ternary complex, with the exception of omitting 5% of the structure during calculation of a composite omit map. Ramachandran statistics for the TCR–SEH–MHC complex were 924 residues (94.48%) in preferred, 42 (4.29%) in allowed and 12 residues in (1.23%) disallowed regions. For the SEH–TCR complex, these statistics were 582 (95.25%), 23 (3.76%) and 6 (0.98%), respectively. Calculations of buried surface areas between proteins in the two complexes were calculated using ArealMol in the CCP4 suite [36] . All protein figures have been produced using PyMol [42] , and structural alignment of the structurally determined SAgs was performed using PROMALS3D [43] . NMR analysis Increasing amount of TCR (JM22:TRAV27/TRVB19) was added to 15 N-labelled SEH and 2D ( 1 H, 15 N) HSQC was recorded at 318 K. Starting concentration of 15 N SEH was 165 μM, and to this sample unlabelled TCR was added to a final concentration of 8 μM, 14 μM and 21 μM, resulting in SEH:TCR ratios of 20:1, 10:1 and 6:1. Sequential assignment of SEH is reported elsewhere, BMRB code 16141 (ref. 20 ). Chemical shifts changes in 1 H and 15 N were weighted together as where Δ 1 H and Δ 15 N are in ppm. The line broadening was evaluated as decrease in peak intensity. The relative peak intensities were normalized to the mean value of each spectrum. The intensity changes induced by the titration were calculated using the following formula. where I 0 and I 21 stand for normalized peak intensities in the spectra of free SEH and added 21 μM TCR, respectively. SEH residues were sorted in accordance with the scores for peak shifts and intensity changes. Residues exhibiting top 20% score in either shift or intensities are given in the Supplementary Table S2 and depicted in Figure 5 . All NMR data were recorded on a Varian 900 MHz Discovery NMR spectrometer equipped with a cold probe. All data were processed in NMRPipe [44] and analyzed using CCPN [45] Accession codes RCSB Protein Data Bank: Coordinates for TCR–SEH–MHC and SEH–TCR structures have been deposited with accession codes 2XN9 and 2XNA , respectively. How to cite this article : Saline, M. et al . The structure of superantigen complexed with TCR and MHC reveals novel insights into superantigenic T cell activation. Nat. Commun. 1:119 doi: 10.1038/ncomms1117 (2010).